Structural and functional characterization of two alpha-synuclein strains α-synuclein aggregation is implicated in a variety of diseases including Parkinson’s disease, dementia with Lewy bodies, pure autonomic failure and multiple system atrophy. The association of protein aggregates made of a single protein with a variety of clinical phenotypes has been explained for prion diseases by the existence of different strains that propagate through the infection pathway. Here we structurally and functionally characterize two polymorphs of α-synuclein. We present evidence that the two forms indeed fulfil the molecular criteria to be identified as two strains of α-synuclein. Specifically, we show that the two strains have different structures, levels of toxicity, and in vitro and in vivo seeding and propagation properties. Such strain differences may account for differences in disease progression in different individuals/cell types and/or types of synucleinopathies. Alzheimer’s, Parkinson’s, Creutzfeldt–Jacob and Huntington’s disease are neurological human proteinopathies intimately linked to the intra- or extra-cellular deposition of megaDalton protein assemblies [1] , [2] . In Parkinson’s disease, which is the second most frequent neurodegenerative disease in humans, the aggregation of alpha-synuclein (α-syn) into fibrillar assemblies in nerve cells is a molecular hallmark of the disease. The aggregates are termed Lewy bodies and Lewy neurites [2] , [3] . α-syn, the major constituent of the aggregates, is a 140-residue presynaptic protein normally found in both soluble and membrane-associated fractions of the brain [4] , [5] . α-syn is believed to have an important role in the regulation of synaptic vesicle release and trafficking, fatty acid-binding and neuronal survival [6] . In vitro , under physiological conditions, α-syn assembles into aggregates that are structurally similar to those found in the inclusions of disease-affected brains. Metastable prefibrillar intermediates form during assembly [7] . These prefibrillar oligomeric species have been reported to be toxic to cells [8] , [9] , [10] . However, we recently demonstrated that α-syn fibrillar assemblies exhibit a level of cytotoxicity at least 1,000-fold higher than that of their precursors at identical particles concentrations [11] . Recent findings suggest that amyloids associated with neurodegenerative diseases spread in a prion-like fashion [12] , [13] , [14] . In a manner akin to prion protein (PrP) aggregation and amplification, fibrillar α-syn assemblies seed the aggregation of monomeric α-syn in vitro [15] , [16] , [17] and spread from one cell to another in cell cultures and animal models [18] , [19] , [20] . In addition, Lewy bodies and Lewy neurites have been shown to spread from the brain of patients developing Parkinson’s disease to grafted neuronal cells [21] , [22] and the intracerebral injection of brain homogenates within the brain of recipient animals has been shown to lead to insoluble α-syn deposits in the CNS and motor symptoms including bradykinesia and rigidity [23] , [24] . Finally, the lesions associated with Parkinson’s disease appear to progress along defined patterns [25] . If these observations point to a prion-like behaviour of α-syn, a typical hallmark of prion diseases has not yet been described for other neurodegenerative illnesses: the presence of strains. Indeed, for prion diseases, a variety of strains that are distinguishable by the disease incubation time in recipient animals, the lesions patterns they cause in the brain and the proteolytic cleavage profiles reflecting structural differences have been described [26] . These strains are believed to be the consequence of different conformations PrP can adopt within its high-molecular weight assemblies that are imprinted to the newly incorporated PrP upon assemblies growth as demonstrated for the yeast prion Sup35p (refs 27 , 28 ). Although A-beta 1–40 fibrils that differ structurally and propagate in test tubes have been generated under slightly different growth conditions resembling that of prion strains [29] , no demonstration of in vivo propagation of these assemblies has been made. Similarly, assemblies made of identical precursor α-syn have not yet been shown to yield specific ‘strains’ that differ by the packing of the protein within the assemblies, the assemblies nucleation propensity, their physical properties, their ability to cross the species barrier, the physiopathological patterns they induce and their incubation time preceding disease onset and recipient animal survival rate as for PrP. Thus, it is not yet clear whether α-syn assemblies possess all the characteristics of infectious prions. In the present work, we generate two different high-molecular weight assemblies from the same precursor α-syn, and characterize their structural behaviour, toxicity and propagation properties. We demonstrate here that each α-syn polymorph propagates faithfully its intrinsic structure in vitro . We also show that the two α-syn polymorphs exhibit marked differences in their propensities to bind and penetrate cells, their toxicity and seeded aggregation of reporter α-syn aggregation in vivo . Finally, we demonstrate that each α-syn polymorph imprints its intrinsic architecture to endogenous reporter α-syn upon its recruitment in vivo . This yields α-syn aggregates within the cells that persist to different extents. Our bottom-up approach suggests that strains can indeed be the molecular origin of different α-synucleinopathies. Structural characterization of two α-syn polymorphs α-syn assembles in vitro into heterogeneous high-molecular weight structures [30] , [31] . This polymorphism reflects the ability of soluble α-syn to populate multiple conformational states that coalesce into distinct high-molecular weight assemblies that grow by incorporation of a given conformational state. We assessed the effect of different assembly conditions on the formation of fibrillar α-syn. In the presence of physiological salt concentrations (buffer A: 50 mM Tris–HCl, pH 7.5, 150 mM KCl) monomeric ( Supplementary Fig. S1 ) α-syn (100 μM) readily assembles within hours, whereas the lag phase preceding assembly takes several days under lower salt concentrations (buffer B: 5 mM Tris-HCl, pH 7.5) ( Fig. 1a ) or in buffer A supplemented with 2.5 mM EDTA ( Supplementary Fig. S2 ). In addition, while the assemblies generated in buffer A depolymerize upon incubation at 4 °C ( Fig. 1b ) and repolymerize upon incubation at 37 °C ( Supplementary Fig. S3 ), those generated in buffer B ( Fig. 1b ) or in buffer A supplemented with 2.5 mM EDTA ( Supplementary Fig. S2 ) are irreversible. 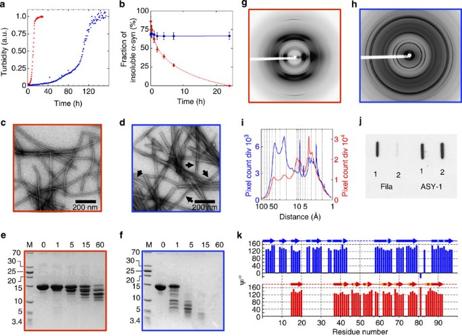Figure 1: Structural characterization of the two α-syn polymorphs. (a) Time courses of α-syn (100 μM) assembly in buffer A (50 mM Tris-HCl, pH 7.5, 150 mM KCl), red data points, and B (5 mM Tris-HCl, pH 7.5), blue data points, at 37 °C, monitored by measurement of scattered light at 440 nm. (b) Time courses of depolymerization at 4 °C of α-syn (100 μM monomer concentration) assemblies obtained in buffer A (high salt, red curve) and B (low salt, blue curve) assessed by quantifying α-syn within the pellet and supernatant fractions by SDS–PAGE, as described in the Methods. Data are mean±s.d. (n=4). (c,d) Negatively stained TEM of α-syn fibrils (c) and ribbons (d). The arrowheads point to twists; scale bars, 200 nm. (e,f), Proteinase K degradation patterns of α-syn (100 μM monomer concentration) fibrils (e) and ribbons (f), monitored over time on Coomassie stained SDS–PAGE (15%). Time (min) and molecular weight markers (kDa) are shown on the top and left of each gel, respectively. (g,h), X-ray diffraction pattern of partially aligned α-syn fibrils (g) and ribbons (h). α-syn fibrils X-ray scattering pattern is typical of amyloids showing a sharp anisotropic reflection at 4.7 Å along the meridian and another anisotropic reflection at 10 Å along the equator while that of α-syn ribbons resembles a powder/crystalline diffraction pattern with sharp meridional and equatorial reflections at 4.75 and 11 Å as well as long- and short-range reflections. (i) Radial averaging of the X-ray scattering patterns of α-syn fibrils (red curve) and ribbons (blue curve). (j) The conformational FILA antibody distinguishes equal amounts (0.4 μg) of α-syn fibrils (1) from α-syn ribbons (2) spotted on nitrocellulose membranes, whereas pan-α-syn antibodies (ASY1) do not. (k) Backbone Ψ angles as predicted by TALOS for α-syn fibrils (red) and ribbons (blue) based on sequential assignment. Suggested ß-sheet are indicated by arrows, with the lighter colours used for extensions if the glycines are assumed to be part of the ß-sheet or when uncertain TALOS β-sheet predictions (marked by crosses) are included into ß-sheets. Some residues in α-syn fibril show slight peak doubling. This is not considered here, as the resulting backbone angles are very similar. Figure 1: Structural characterization of the two α-syn polymorphs. ( a ) Time courses of α-syn (100 μM) assembly in buffer A (50 mM Tris-HCl, pH 7.5, 150 mM KCl), red data points, and B (5 mM Tris-HCl, pH 7.5), blue data points, at 37 °C, monitored by measurement of scattered light at 440 nm. ( b ) Time courses of depolymerization at 4 °C of α-syn (100 μM monomer concentration) assemblies obtained in buffer A (high salt, red curve) and B (low salt, blue curve) assessed by quantifying α-syn within the pellet and supernatant fractions by SDS–PAGE, as described in the Methods. Data are mean±s.d. ( n =4). ( c , d ) Negatively stained TEM of α-syn fibrils ( c ) and ribbons ( d ). The arrowheads point to twists; scale bars, 200 nm. ( e , f ), Proteinase K degradation patterns of α-syn (100 μM monomer concentration) fibrils ( e ) and ribbons ( f ), monitored over time on Coomassie stained SDS–PAGE (15%). Time (min) and molecular weight markers (kDa) are shown on the top and left of each gel, respectively. ( g , h ), X-ray diffraction pattern of partially aligned α-syn fibrils ( g ) and ribbons ( h ). α-syn fibrils X-ray scattering pattern is typical of amyloids showing a sharp anisotropic reflection at 4.7 Å along the meridian and another anisotropic reflection at 10 Å along the equator while that of α-syn ribbons resembles a powder/crystalline diffraction pattern with sharp meridional and equatorial reflections at 4.75 and 11 Å as well as long- and short-range reflections. ( i ) Radial averaging of the X-ray scattering patterns of α-syn fibrils (red curve) and ribbons (blue curve). ( j ) The conformational FILA antibody distinguishes equal amounts (0.4 μg) of α-syn fibrils (1) from α-syn ribbons (2) spotted on nitrocellulose membranes, whereas pan-α-syn antibodies (ASY1) do not. ( k ) Backbone Ψ angles as predicted by TALOS for α-syn fibrils (red) and ribbons (blue) based on sequential assignment. Suggested ß-sheet are indicated by arrows, with the lighter colours used for extensions if the glycines are assumed to be part of the ß-sheet or when uncertain TALOS β-sheet predictions (marked by crosses) are included into ß-sheets. Some residues in α-syn fibril show slight peak doubling. This is not considered here, as the resulting backbone angles are very similar. Full size image Transmission electron microscopy (TEM) reveals that while the assemblies generated buffer A have a cylindrical aspect ( Fig. 1c ), those obtained under lower salt conditions ( Fig. 1d ) or in buffer A supplemented with 2.5 mM EDTA ( Supplementary Fig. S2 ) are flat. In contrast to the cylindrical polymers, the flat assemblies often twist (arrowheads in Fig. 1d ), as do ribbons. The cylindrical and flat natures of the assemblies were further assessed by cryo-electron microscopy. Supplementary Figure S4 shows that while the cylindrical fibrils have a constant width (13±2 nm s.e.m., n =50), the flat fibrils twist with alternating wide (white arrowheads, 18±1.5 nm s.e.m., n =50) and narrow (black arrowheads, 8±1 nm s.e.m., n =50) sections. We will therefore refer to the cylindrical assemblies as α-syn fibrils and to the flat, twisting assemblies as α-syn ribbons. Limited proteolysis of α-syn fibrils and ribbons over time reveals substantial differences, as shown for proteinase K digestion in Fig. 1e,f , respectively. Full-length α-syn resists proteinase K treatment for up to 60 min within the fibrils, and five major polypeptides with apparent molecular masses ranging from 14 to 11 kDa are generated ( Fig. 1e ). In contrast, full-length α-syn in ribbons is fully degraded in <5 min and polypeptides with apparent molecular weight ranging from 10 to 4 kDa are generated ( Fig. 1f ). The Fourier transform infrared (FTIR) spectra of α-syn fibrils and α-syn ribbons ( Supplementary Fig. S5 ) and their deconvolution indicate that the ß-sheet content of α-syn ribbons (79.5%) is slightly higher than that of α-syn fibrils (75.2%) ( Table 1 ). In agreement with their high ß-sheet content, both assemblies bind Congo red and exhibit the yellow green birefringence that is considered as a hallmark of amyloids ( Supplementary Fig. S6A ). Interestingly, however, at identical amounts of assembled α-syn ( Supplementary Fig. S6B ), α-syn fibrils were found to bind Thioflavin T, whereas α-syn ribbons did not ( Supplementary Fig. S6C ). Table 1 FTIR deconvolution. Full size table X-ray fibre diffraction measurements on partially aligned α-syn fibrils ( Fig. 1g ) and α-syn ribbons ( Fig. 1h ) differ very significantly. The pattern in Fig. 1g resembles the pattern of amyloids, with an intense and characteristic anisotropic reflection at 4.7±0.2 Å, s.d., spacing along the meridian and another anisotropic reflection at 10±0.2 Å, s.d., spacing along the equator. Strong cross-peaks at 3.7±0.2 Å, s.d., that are neither meridional nor equatorial are also visible. Similarly, long-range reflections at 44 and 22.7±0.8 Å, s.d., indicative of the unit cell size were observed. In contrast, the X-ray scattering pattern from α-syn ribbons ( Fig. 1h ) resembles a powder/crystalline diffraction pattern, containing sharp meridional and equatorial reflections at 4.75±0.05, s.d., and 11±0.1 Å, s.d., also long and short-range reflections. The diffraction limit of α-syn fibrils is 1.236 Å and that for α-syn ribbons is 1.12. The radial averaging of the X-ray scattering patterns of α-syn fibrils and ribbons are overlayed in Fig. 1i . The long-range reflections for ribbons are different from those we measured for α-syn fibrils, suggesting that the unit cell in α-syn ribbons differs from that in α-syn fibrils. Most interesting, the short-range reflections in α-syn ribbons are very sharp. This indicates that the correlation length within α-syn ribbons (300 Å) is much higher than in α-syn fibrils (100 Å), for example, the ribbons are crystalline-like with a very high long-range order as opposed to the fibrils. The reflections, orientation and the tentative hkl assignment are given in Supplementary Tables S1 and S2 for α-syn fibrils and ribbons, respectively. The size of the unit cell can be derived from the reflections as 44.04 × 22.77 × 4.66 Å for α-syn fibrils and 44.6 × 42.02 × 4.75 Å for α-syn ribbons. We next assessed differences in the conformation of α-syn molecules within α-syn fibrils and ribbons using the FILA-1 conformational antibody that recognizes specifically α-syn fibrils [32] . Figure 1j shows that FILA-1 antibody recognizes α-syn fibrils but not equal amounts (400 ng) of α-syn ribbons spotted on nitrocellulose filters. This indicates that the epitope exposed to the solvent in α-syn fibrils is not in the ribbons. Solid-state NMR measurements elucidate the structural differences between the two polymorphs on a residue-per-residue basis. Such measurements allowed correlating differences in α-syn fibrils morphologies with differences in molecular structures [33] . We recorded solid-state NMR spectra from α-syn ribbons and α-syn fibrils. Both feature narrow lines ( Supplementary Fig. S7 ). This indicates that α-syn ribbons and fibrils samples are homogeneous in the sense that they consist of a single, well-defined polymorph. NMR secondary chemical shifts, which are sensitive indicators of secondary structure, were derived from the sequential resonance assignment of the two forms by three-dimensional (3D) spectroscopy. We assigned both α-syn ribbons [34] and fibrils [35] spectra, none of which coincided with published data on α-syn fibrillar assemblies [33] , [36] , [37] , [38] . The backbone chemical shifts are very sensitive to the backbone dihedral angles and can be used to predict those angles and consequently the secondary structure elements. Figure 1k shows the Ψ backbone angles for fibrils and ribbons as predicted by TALOS (ref. 39 ). The number and position of predicted β-sheet, loop and turn of secondary structure elements reported by others [33] , [36] differ from those we report for the two polymorphs we generated. In addition, while the region spanning α-syn residues 1–38 appears unstructured in all previously generated polymorphs, the entire N-terminal part of the protein, down to residue 1, is rigid and ordered into β-sheets in α-syn ribbons and the region spanning residues 16–20 adopts β-sheet structure in α-syn fibrils. The two polymorphs display β-sheet structure. However, the distribution of the secondary structure elements within α-syn ribbons and fibrils is very different. The N-terminal part of α-syn ribbons predominantly forms a rigid β-sheet, whereas the N-terminal part of the fibrils is largely disordered (static and/or dynamic disorder), with the notable exception of a short stretch. Overall, 83 amino acid residues spanning residues 1–43 and 58–97 in α-syn ribbons as opposed to 61 amino acid residues spanning residues 16–20 and 38–92 in α-syn fibrils form highly ordered structures. Our finding that the N terminus has a role in α-syn fibrils and ribbons structural organization contrasts with earlier suggestions where the first thirty residues were described as flexible/dynamic and solvent-exposed [40] , [41] , [42] . α-syn fibrils did not convert into ribbons in buffer B or buffer A containing EDTA and α-syn ribbons did not convert into fibrils in buffer A upon incubation for 60 days at room temperature. This indicates that the two polymorphs do not interconvert in their assembled forms. Altogether, the results of this broad range of structural and biochemical measurements unequivocally demonstrate that α-syn molecules adopt different conformations and are arranged in a different manner in α-syn fibrils and α-syn ribbons, even though both forms consists predominantly of ß-sheets. Propagation of the two α-syn polymorphs in vitro The efficiency with which preformed fibrils elongate reflects their capacity to recruit monomers and imprint their intrinsic structure to the soluble precursor proteins. Thus, differences in the intrinsic architecture of two polymorphs should reflect in their ability to elongate. We measured the nucleation capacities of α-syn fibrils and ribbons under different experimental conditions and examined the nature of the polymers that form by TEM and limited proteolysis. The lag phase preceding assembly is abolished upon seeding soluble α-syn assembly by α-syn fibrils in buffer A ( Fig. 2a ) and the polymers that form are fibrils. Seeding with α-syn ribbons under the same experimental conditions also abolishes the lag phase preceding assembly. Surprisingly however, given that ribbons do not form spontaneously in buffer A, the polymers that are generated are of a ribbon nature as revealed by TEM and limited proteolysis. In contrast, α-syn ribbons are generated irrespective of the nature of the seeds, fibrils or ribbons added to soluble α-syn in buffer B ( Fig. 2b ). Our findings clearly indicate that α-syn fibrils and ribbons imprint intrinsic architecture to soluble α-syn molecules upon their recruitment and incorporation within fibrils or ribbons in buffer A. This also suggests that the two polymorphs propagate structural information. The finding that fibrils seed the formation of α-syn ribbons in buffer B suggests that soluble α-syn does not sample the conformation(s) that sustain α-syn fibrils elongation, for example, that incorporate into α-syn fibrils, while the folding intermediates that form ribbons are populated. 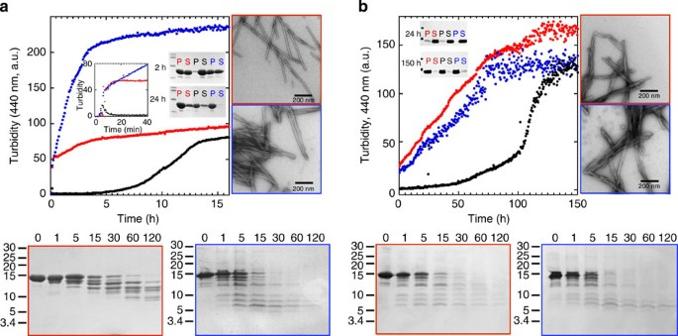Figure 2: Cross-seeding capacities of the two α-syn polymorphs. Elongation of preformed α-syn fibrils (red data points) and ribbons (blue data points), 10 μM in (a) buffer A (50 mM Tris-HCl, pH 7.5, 150 mM KCl), (b) buffer B (5 mM Tris-HCl, pH 7.5), at 37 °C, in the presence of soluble α-syn (100 μM), monitored by measurement of scattered light at 440 nm. The control assembly reactions of soluble α-syn in the absence of preformed seeds (black data points) are also shown. When the seeded assembly reactions were centrifuged immediately after addition of the seeds (40,000gfor 30 min at 20 °C) and the supernatant and pellet fractions analysed by SDS–PAGE, the pellets contained the added seeds (fibrils or ribbons, 10% of the protein), whereas the supernatants contained the soluble α-syn (90% of the protein content of the solution). The amount of α-syn in the pellet and supernatant fractions at the indicated time (2, 24 and 150 h) in the absence (black letters) or the presence of α-syn fibrils (red letters) and ribbons (blue letters) seeds revealed by Coomassie blue stained SDS–PAGE are also shown. The inset in (a) corresponds to a blow-up on the initial stages of the assembly reactions. Electron micrographs and SDS–PAGE proteinase K degradation patterns of α-syn assemblies generated upon addition of preformed α-syn fibrils and ribbons are shown. The time (in min) and molecular weight markers (in kDa) are shown on the top and left of each Coomassie blue stained SDS–PAGE. The scale bars in the electron micrographs correspond to 200 nm. Figure 2: Cross-seeding capacities of the two α-syn polymorphs. Elongation of preformed α-syn fibrils (red data points) and ribbons (blue data points), 10 μM in ( a ) buffer A (50 mM Tris-HCl, pH 7.5, 150 mM KCl), ( b ) buffer B (5 mM Tris-HCl, pH 7.5), at 37 °C, in the presence of soluble α-syn (100 μM), monitored by measurement of scattered light at 440 nm. The control assembly reactions of soluble α-syn in the absence of preformed seeds (black data points) are also shown. When the seeded assembly reactions were centrifuged immediately after addition of the seeds (40,000 g for 30 min at 20 °C) and the supernatant and pellet fractions analysed by SDS–PAGE, the pellets contained the added seeds (fibrils or ribbons, 10% of the protein), whereas the supernatants contained the soluble α-syn (90% of the protein content of the solution). The amount of α-syn in the pellet and supernatant fractions at the indicated time (2, 24 and 150 h) in the absence (black letters) or the presence of α-syn fibrils (red letters) and ribbons (blue letters) seeds revealed by Coomassie blue stained SDS–PAGE are also shown. The inset in ( a ) corresponds to a blow-up on the initial stages of the assembly reactions. Electron micrographs and SDS–PAGE proteinase K degradation patterns of α-syn assemblies generated upon addition of preformed α-syn fibrils and ribbons are shown. The time (in min) and molecular weight markers (in kDa) are shown on the top and left of each Coomassie blue stained SDS–PAGE. The scale bars in the electron micrographs correspond to 200 nm. Full size image Toxicity of the two α-syn polymorphs To compare the relative toxicities of α-syn fibrils and ribbons at similar particle concentrations, we generated α-syn fibrils and ribbons of identical length (as demonstrated by quantitative TEM and length distribution measurements in Supplementary Fig. S8 ) and determined the average number of α-syn molecules in the two forms of the protein using analytical centrifugation as described [11] . We find that ribbons and fibrils are formed by 800 and 7,000 monomers on average, respectively (see the Methods section and Supplementary Fig. S8 ). The cytotoxicity of equal particle concentrations of α-syn fibrils and ribbons was assessed on human neuroblastoma SH-SY5Y cells using cell survival counting and the 3-(4,5-dimethylthiazol-2-yl)-2,5-diphenyltetrazolium bromide (MTT) assay ( Fig. 3a,b ). Fibrillar α-syn appeared more toxic to the cells than α-syn ribbons as assessed by cell survival counting after lifting the cells by EDTA, incubating them in the presence of increasing concentrations of α-syn fibrils or ribbons, replating and counting them after 24 h in the presence of trypan blue ( Fig. 3a ). Assessment of cell survival using the MTT assay ( Fig. 3b ) shows a similarity in trend with the differences detected using the cell viability assay. We conclude from these observations that α-syn fibrils are more toxic to cells than α-syn ribbons. In agreement with the latter, α-syn fibrils induced the activation of caspase-3 in a concentration-dependent manner to a higher extent than α-syn ribbons ( Fig. 3c ), suggesting that they are more efficient in triggering apoptotic cell death than α-syn ribbons. 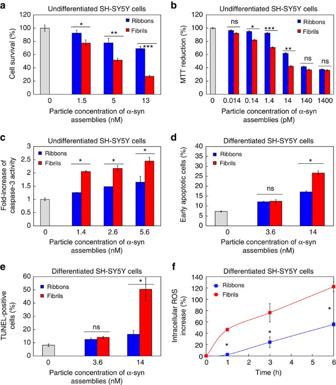Figure 3: Toxicity of the two α-syn polymorphs. Viability of undifferentiated SH-SY5Y cells treated for 24 h with increasing particle concentrations of α-syn fibrils (red bars) and ribbons (blue bars), measured by (a) cell survival counting and (b) MTT assay. Control cells treated with assembly buffer (grey bars) are shown. Data foraandbare mean±s.e. (n=6 independent measurements) expressed as percentages relative to controls. Ribbons versus fibrils, *P<0.05; **P<0.01; ***P<0.001 (two-sample, two-tailed independent Student’st-test). (c) Caspase-3 activation in SH-SY5Y cells treated for 24 h with increasing particle concentrations of α-syn fibrils (red bars) and ribbons (blue bars). Data are shown as fold increase relative to the caspase-3 activity measured in control cells treated with assembly buffer (grey bar). Data are mean±s.e. (n=3 independent measurements). Ribbons versus fibrils, *P<0.05 (two-sample, two-tailed independent Student’st-test). Increase in annexin V-PE labelling, (d) and DNA fragmentation, (e) upon treatment of differentiated SH-SY5Y cells with increasing particle concentrations of α-syn fibrils (red bars) and ribbons (blue bars) for 48 h. Control differentiated cells treated with buffer are also shown (grey bars). Annexin V-PE labelling data are percentages of annexin V-PE-positive/7-AAD-negative cells (early apoptotic cells) obtained from three independent experiments. Error bars are denoted as s.e. Ribbons versus fibrils, *P<0.05 (two-sample, two-tailed independent Student’st-test). In the DNA fragmentation measurements, data are percentages of TUNEL-positive cells obtained from three independent experiments. Error bars are denoted as s.e. Ribbons versus fibrils, *P<0.05 (two-sample, two-tailed independent Student’st-test) with control cells treated with assembly buffer. (f) Time course of intracellular ROS levels increase in differentiated SH-SY5Y cells treated with α-syn fibrils (red curve) and ribbons (blue curve), 0.2 nM. Cells were loaded with CellROX Orange Reagent and imaged by epifluorescence microscopy (see alsoSupplementary Fig. S8). Data are shown as percentage increase relative to the fluorescence values measured at time 0 (control untreated cells). Data are mean±s.e. (n=3 independent measurements). Ribbons versus fibrils, *P<0.05 (two-sample, two-tailed independent Student’st-test). Figure 3: Toxicity of the two α-syn polymorphs. Viability of undifferentiated SH-SY5Y cells treated for 24 h with increasing particle concentrations of α-syn fibrils (red bars) and ribbons (blue bars), measured by ( a ) cell survival counting and ( b ) MTT assay. Control cells treated with assembly buffer (grey bars) are shown. Data for a and b are mean±s.e. ( n =6 independent measurements) expressed as percentages relative to controls. Ribbons versus fibrils, * P <0.05; ** P <0.01; *** P <0.001 (two-sample, two-tailed independent Student’s t -test). ( c ) Caspase-3 activation in SH-SY5Y cells treated for 24 h with increasing particle concentrations of α-syn fibrils (red bars) and ribbons (blue bars). Data are shown as fold increase relative to the caspase-3 activity measured in control cells treated with assembly buffer (grey bar). Data are mean±s.e. ( n =3 independent measurements). Ribbons versus fibrils, * P <0.05 (two-sample, two-tailed independent Student’s t -test). Increase in annexin V-PE labelling, ( d ) and DNA fragmentation, ( e ) upon treatment of differentiated SH-SY5Y cells with increasing particle concentrations of α-syn fibrils (red bars) and ribbons (blue bars) for 48 h. Control differentiated cells treated with buffer are also shown (grey bars). Annexin V-PE labelling data are percentages of annexin V-PE-positive/7-AAD-negative cells (early apoptotic cells) obtained from three independent experiments. Error bars are denoted as s.e. Ribbons versus fibrils, * P <0.05 (two-sample, two-tailed independent Student’s t -test). In the DNA fragmentation measurements, data are percentages of TUNEL-positive cells obtained from three independent experiments. Error bars are denoted as s.e. Ribbons versus fibrils, * P <0.05 (two-sample, two-tailed independent Student’s t -test) with control cells treated with assembly buffer. ( f ) Time course of intracellular ROS levels increase in differentiated SH-SY5Y cells treated with α-syn fibrils (red curve) and ribbons (blue curve), 0.2 nM. Cells were loaded with CellROX Orange Reagent and imaged by epifluorescence microscopy (see also Supplementary Fig. S8 ). Data are shown as percentage increase relative to the fluorescence values measured at time 0 (control untreated cells). Data are mean±s.e. ( n =3 independent measurements). Ribbons versus fibrils, * P <0.05 (two-sample, two-tailed independent Student’s t -test). Full size image To further assess the effect of α-syn fibrils or ribbons on cells, early and late apoptotic markers were measured. Co-labelling of differentiated SH-SY5Y cells with phycoerythrin-labelled annexin V (annexin V-PE) and 7-amino-actinomycin D (7-AAD) revealed a concentration-dependent increase in annexin V-PE-positive cells after treatment for 48 h with α-syn polymorphs ( Fig. 3d ), whereas the increase in 7-AAD labelling was negligible (3±1%, s.e.m., n =3 independent measurements), indicating that treated cells undergo apoptotic rather than necrotic death. Accordingly, an increase in nuclear DNA fragmentation ( Fig. 3e and Supplementary Fig. S9 ) was observed in differentiated SH-SY5Y cells within 48 h. In addition and in agreement with the finding that α-syn fibrils are more toxic than ribbons, the level of both apoptotic markers was significantly higher in the presence of α-syn fibrils. Finally, we measured oxidative stress by monitoring intracellular reactive oxygen species (ROS) levels over time upon exposure of differentiated SH-SY5Y cells to α-syn fibrils or ribbons. Figure 3f and Supplementary Fig. S10 show that ROS levels are significantly higher in cells exposed for 1–6 h to α-syn fibrils as compared with α-syn ribbons. Altogether these observations strongly suggest that α-syn fibrils and ribbons differ functionally, with α-syn fibrils inducing to a much higher extent biochemical modifications within the cells that trigger the apoptotic pathway, eventually leading to cell death by apoptosis rather than by necrosis. Functional properties of the two α-syn polymorphs We recently showed that the cytotoxicity associated with α-syn fibrils is the consequence of their binding and permeabilization of membrane lipid bilayers [11] . We therefore assessed the membrane-binding properties of the two α-syn polymorphs using an ultracentrifugation floatation assay. We found that α-syn ribbons (8 nM) bind to artificial lipid vesicles to a higher extent and are found in higher amounts in the top fractions (fractions 1–4) of the gradient when mixed with 6.25 mM vesicles of 1,2-dioleoyl phosphatidylcholine (DOPC), 1,2-dioleoyl phosphatidylserine (DOPS) or 1,2-dioleoyl phosphatidylglycerol (DOPG) (blue bars in Fig. 4a–c ), as compared with equivalent concentrations of α-syn fibrils of identical length (red bars in Fig. 4a–c ). α-syn fibrils and ribbons bound equally well to complex lipid mixtures extracted from porcine brain ( Fig. 4d ). We then assessed membrane integrity and permeability following binding of α-syn fibrils and ribbons using a calcein release assay. Unilamellar vesicles with different compositions were prepared in the presence of calcein (60 mM), and calcein release upon the addition of α-syn (0.7 nM) fibrils or ribbons was monitored over time. Somewhat surprisingly, given their lower lipid vesicle-binding capacity, α-syn fibrils permeabilized lipid vesicles made of DOPS and DOPG to a much higher extent as judged from the fluorescence increase recorded by us compared with equivalent concentrations of α-syn ribbons ( Fig. 4e–g ). 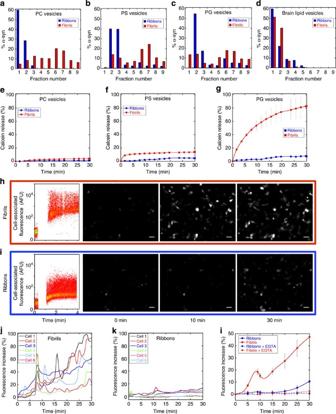Figure 4: Differential interaction of the two α-syn polymorphs with synthetic and cell membranes. Binding of 8 nM α-syn fibrils (red bars) and ribbons (blue bars) to (a) DOPC, (b) DOPS, (c) DOPG and (d) lipid extracts from brain unilamellar vesicles (6.25 mM lipids) measured by flotation. Membrane-bound α-syn assemblies were separated from free α-syn assemblies by density gradient ultracentrifugation. Data represent the distribution of α-syn fibrils (red bars) and ribbons (blue bars) in the different fractions of the density gradient, quantified by SDS–PAGE. Increasing fraction numbers on thexaxes correspond to increasing densities. Calcein release from (e) DOPC, (f) DOPS and (g) DOPG unilamellar vesicles induced by 0.7 nM α-syn fibrils (red bars) and ribbons (blue bars). The α-syn assemblies were added to calcein-loaded vesicles and the fluorescence measured for 30 min. The data are obtained by subtracting the percentage of spontaneous calcein release measured in control vesicles treated with identical volumes of assembly buffer. Data are denoted as mean±s.e. (n=3 independent measurements). Time-dependent α-syn fibrils, (h), and ribbons, (i), binding to cells and increase in intracellular Ca2+levels. Binding of 0.1 nM Alexa Fluor 488-labelled α-syn polymorphs to SH-SY5Y cells (left panels) was assessed by flow cytometry. The measurement dead time is 20 s. Cells loaded with Fluo-4-AM were imaged by epifluorescence microscopy after exposure to the two α-syn polymorphs to assess alterations in intracellular free Ca2+levels. Scale bars, 30 μm. Quantification of the intracellular free Ca2+increase measured over time for all the duration of the experiment in six representative cells exposed to α-syn fibrils (j) or ribbons (k), expressed as a fraction of the fluorescence recorded upon addition of ionomycin (10 μM) to the cells. (l) Kinetics of the intracellular free Ca2+variation induced by α-syn fibrils (red curves) or ribbons (blue curves) in the absence (solid lines) or the presence of 5 mM EGTA (dashed lines). Data are mean±s.e. of the fluorescence measured in 50 different cellular areas of 20 μm2each. Figure 4: Differential interaction of the two α-syn polymorphs with synthetic and cell membranes. Binding of 8 nM α-syn fibrils (red bars) and ribbons (blue bars) to ( a ) DOPC, ( b ) DOPS, ( c ) DOPG and ( d ) lipid extracts from brain unilamellar vesicles (6.25 mM lipids) measured by flotation. Membrane-bound α-syn assemblies were separated from free α-syn assemblies by density gradient ultracentrifugation. Data represent the distribution of α-syn fibrils (red bars) and ribbons (blue bars) in the different fractions of the density gradient, quantified by SDS–PAGE. Increasing fraction numbers on the x axes correspond to increasing densities. Calcein release from ( e ) DOPC, ( f ) DOPS and ( g ) DOPG unilamellar vesicles induced by 0.7 nM α-syn fibrils (red bars) and ribbons (blue bars). The α-syn assemblies were added to calcein-loaded vesicles and the fluorescence measured for 30 min. The data are obtained by subtracting the percentage of spontaneous calcein release measured in control vesicles treated with identical volumes of assembly buffer. Data are denoted as mean±s.e. ( n =3 independent measurements). Time-dependent α-syn fibrils, ( h ), and ribbons, ( i ), binding to cells and increase in intracellular Ca 2+ levels. Binding of 0.1 nM Alexa Fluor 488-labelled α-syn polymorphs to SH-SY5Y cells (left panels) was assessed by flow cytometry. The measurement dead time is 20 s. Cells loaded with Fluo-4-AM were imaged by epifluorescence microscopy after exposure to the two α-syn polymorphs to assess alterations in intracellular free Ca 2+ levels. Scale bars, 30 μm. Quantification of the intracellular free Ca 2+ increase measured over time for all the duration of the experiment in six representative cells exposed to α-syn fibrils ( j ) or ribbons ( k ), expressed as a fraction of the fluorescence recorded upon addition of ionomycin (10 μM) to the cells. ( l ) Kinetics of the intracellular free Ca 2+ variation induced by α-syn fibrils (red curves) or ribbons (blue curves) in the absence (solid lines) or the presence of 5 mM EGTA (dashed lines). Data are mean±s.e. of the fluorescence measured in 50 different cellular areas of 20 μm 2 each. Full size image We next investigated the consequences of the interaction of α-syn fibrils and ribbons (6 nM) with the cell membranes. As demonstrated previously, fluorescently labelled fibrillar α-syn bound efficiently to the plasma membranes of cultured SH-SY5Y cells [11] . Binding was rapid (with saturation within 120 s), as assessed by monitoring Alexa Fluor 488-labelled α-syn fibrils using flow cytometry ( Fig. 4h , left panel). Binding of α-syn fibrils to the cells induced a progressive increase in intracellular free Ca 2+ over time as assessed by the increase in the fluorescence of SH-SY5Y cells loaded with Fluo-4-acetoxymethyl ester (Fluo-4-AM) ( Fig. 4h,j,l ), whether the measurement was performed on six randomly chosen individual cells ( Fig. 4j ) or on a region with >50 cells ( Fig. 4l ). Although the binding of α-syn ribbons to the cells was as rapid as that of fibrils ( Fig. 4i , left panel), the extent of cell-bound α-syn ribbons was two orders of magnitude lower than that of α-syn fibrils with identical intrinsic fluorescence intensity (compare the left panels in Fig. 4h,i ), indicating that α-syn fibrils bind to cells with higher affinity as compared with α-syn ribbons. In the experiments where α-syn fibrils and ribbons binding to cells was monitored by flow cytometry, the cell population was gated by forward and side scatter and at least 10,000 cells were recorded. The geometric means of the gated population was determined. For cells prior to treatment with ribbons, the values are: counts 3,359/mean, 5.95/s.d. 3.22. For cells treated with ribbons the values are: counts 31,434/mean, 1,674/s.d. 105. For cells prior to treatment with fibrils, the values are: counts 3,098/mean, 3.44/s.d. 4.19. For cells treated with fibrils the values are: counts 27,964/mean, 88.1/s.d. 63.2. Given that ribbons and fibrils bind brain lipid vesicles with similar affinities, the greater binding of fibrils to cells is certainly due to the presence of proteins or receptors within the cell membrane. The amplitude of the intracellular free Ca 2+ levels increase recorded by us was much smaller and the time course of intracellular Ca 2+ increase much slower upon exposure of the cells to α-syn ribbons ( Fig. 4i,k,l ). Neither the cell-to-cell variability nor the rapid bursts of intracellular free Ca 2+ increase observed by us upon exposure of the cells to α-syn fibrils were seen upon addition of α-syn ribbons. To identify Ca 2+ origin, the culture medium was supplemented with 5 mM EGTA and the measurements repeated. No intracellular free Ca 2+ increase was observed upon exposure of the cells to α-syn fibrils or ribbons ( Fig. 4l ). This suggests that the free Ca 2+ influxes originate from the extracellular medium. Altogether, these measurements show that α-syn fibrils bind to and permeabilize cell membranes to a great extent. Propagation of the two α-syn polymorphs in mammalian cells We recently demonstrated the uptake and transport of exogenous α-syn assemblies by cultured cells, including primary neuronal cultures [43] . Externally applied α-syn assemblies reach the cytosol of cultured cells and neurons where they nucleate the polymerization of cytoplasmic α-syn [24] . To assess the nucleation efficiency of the two α-syn polymorphs generated by us, Neuro 2a cells stably expressing ChFP-tagged α-syn (α-syn-ChFP) were exposed to α-syn fibrils or ribbons at identical particle concentrations, and the efficacy of ChFP fluorescence redistributed into distinct foci was monitored over time either in real-time fluorescence microscopy or after fixing the cells. ChFP fluorescence in untreated cells showed a diffuse nucleocytoplasmic distribution as expected for a soluble protein ( Fig. 5e ). This distribution was unaffected when the cells were exposed to fibrillar Huntingtin Exon 1 with 45Q, Aß 1–42 and the yeast prion Sup35 when the cells were exposed to α-syn fibrils (0.01 nM), ChFP fluorescence redistributed into distinct foci ( Fig. 5a ). These foci colocalized extensively with the exogenous Alexa Fluor 488-labelled α-syn fibrils puncta. Quantification of the extent of colocalization indicated that nearly 90% of Alexa Fluor 488 α-syn fibrils puncta coincide with ChFP puncta, suggesting that the intracellular and extracellular proteins had indeed coalesced into common intracellular foci. Conversion of the soluble cytoplasmic reporter α-syn to an insoluble aggregated form is first detectable within 1 h after cell exposure to the exogenous α-syn fibrils (with ~16% of the cells exhibiting ChFP puncta). Over 90% of the cells exhibited ChFP puncta within 4 h ( Fig. 5a ). In contrast, no ChFP puncta could be observed after exposure of the cells to α-syn ribbons (4 h at 0.1 nM, Fig. 5b ), despite the fact that α-syn ribbons bound well and were internalized as efficiently as α-syn fibrils. The first ribbon-induced puncta were observed 18 h after exposure of the cells to α-syn ribbons at higher concentrations (0.1 nM) ( Fig. 5d ). At the same time point, all cells exposed to α-syn fibrils (0.01 nM) had massive puncta ( Fig. 5c ). This indicates that α-syn fibrils have higher nucleating and amplifying activities in vivo as compared with α-syn ribbons. 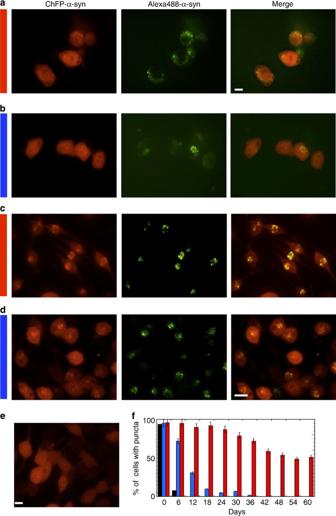Figure 5: Differential seeding properties of the two α-syn polymorphs. The diffuse distribution of ChFP-α-syn fluorescence in Neuro 2a cells (a) was converted to a punctate pattern within 4 h upon exposure of the cells to Alexa Fluor 488-labelled α-syn fibrils (0.01 nM). (b) No such redistribution was observed within the same time frame upon treatment of the cells with α-syn ribbons at a 10 fold higher concentration (0.1 nM). (d) The first ChFP-α-syn puncta were apparent in cells exposed for 18 h to α-syn ribbons (0.1 nM) (c) a time at which ChFP-α-syn was almost entirely recruited into puncta in cells exposed to α-syn fibrils (0.01 nM). (e) control cells unexposed to α-syn fibrils or ribbons. The merged images (right column) show that ChFP-α-syn puncta colocalize extensively with the exogenous Alexa Fluor 488-labelled α-syn polymorphs. Scale bar, 10 μm. (f) Neuro 2a cells exposed 48 h to α-syn fibrils or ribbons (0.1 nM) were passaged 2–3 times a week. The generation time of N2A cells under our experimental conditions was 14–16 h. The presence of internalized aggregates (green fluorescence) and induced puncta (red fluorescence) was scored in a blind manner by two scientists. The time courses of exogenous α-syn fibrils or ribbons (in black) and puncta induced by ribbons (blue) or fibrils (red) disappearance are shown. Data are mean±s.d. (n=3 independent measurements). Figure 5: Differential seeding properties of the two α-syn polymorphs. The diffuse distribution of ChFP-α-syn fluorescence in Neuro 2a cells ( a ) was converted to a punctate pattern within 4 h upon exposure of the cells to Alexa Fluor 488-labelled α-syn fibrils (0.01 nM). ( b ) No such redistribution was observed within the same time frame upon treatment of the cells with α-syn ribbons at a 10 fold higher concentration (0.1 nM). ( d ) The first ChFP-α-syn puncta were apparent in cells exposed for 18 h to α-syn ribbons (0.1 nM) ( c ) a time at which ChFP-α-syn was almost entirely recruited into puncta in cells exposed to α-syn fibrils (0.01 nM). ( e ) control cells unexposed to α-syn fibrils or ribbons. The merged images (right column) show that ChFP-α-syn puncta colocalize extensively with the exogenous Alexa Fluor 488-labelled α-syn polymorphs. Scale bar, 10 μm. ( f ) Neuro 2a cells exposed 48 h to α-syn fibrils or ribbons (0.1 nM) were passaged 2–3 times a week. The generation time of N2A cells under our experimental conditions was 14–16 h. The presence of internalized aggregates (green fluorescence) and induced puncta (red fluorescence) was scored in a blind manner by two scientists. The time courses of exogenous α-syn fibrils or ribbons (in black) and puncta induced by ribbons (blue) or fibrils (red) disappearance are shown. Data are mean±s.d. ( n =3 independent measurements). Full size image We next compared the persistence and propagation that is, the inheritance of the two α-syn isoforms in cells transiently exposed to α-syn fibrils or ribbons. Forty-eight hours after exposure of the cells to the two isoforms, the extracellular assemblies had entered the cells and provoked the coalescence of the otherwise soluble cytosolic and evenly distributed reporter fluorescent α-syn into puncta. The input extracellular assemblies declined over time and were no more detected because of dilution of the initial inoculum following cell division after the 8th generation. However, cells initially exposed to α-syn fibrils had persistent punctate phenotype at the 95th generation for example, 60 days ( Fig. 5f ). In contrast, the fuzzy punctate appearance in cells initially exposed to α-syn ribbons did not persist beyond the 45th generation for example, 30 days ( Fig. 5f ). These findings strongly suggest that endogenous α-syn aggregation that is seeded by extracellular assemblies is a persistent and heritable phenotype, also that the two α-syn polymorphs propagate in vivo with different efficiencies. To demonstrate that the two α-syn polymorphs propagate their intrinsic architectures in vivo upon recruitment of the endogenous α-syn, Neuro 2A stably expressing ChFP-tagged α-syn were exposed to α-syn fibrils (0.2 nM) or ribbons (2.2 nM) for 24 h. The cells were recovered 4 days later, lysed and the cellular lysate subjected to proteolysis in the presence of increasing concentrations of proteinase K. Analysis of the digestion products by SDS–PAGE ( Fig. 6 ) reveals that the degradation pattern of ChFP-tagged α-syn puncta seeded by α-syn fibrils ( Fig. 6a ) differs very significantly from that of ChFP-tagged α-syn puncta seeded by α-syn ribbons ( Fig. 6b ). Both patterns differ from that of ChFP-tagged α-syn from untreated Neuro 2A cells ( Fig. 6c ). We conclude from these observations that exogenous α-syn fibrils and ribbons imprint their intrinsic architecture to endogenous α-syn upon its recruitment in vivo . This, together with the finding that the resulting puncta are heritable and persist to different extent, strongly suggests that the two polymorphs generated by us correspond to distinct α-syn strains. 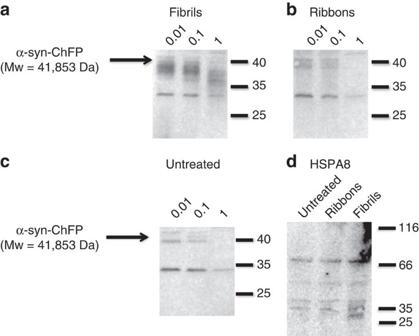Figure 6: The two α-syn polymorphs imprint their intrinsic architecture to endogenous α-syn upon its recruitment. Western blot analysis of the degradation profiles of the reporter ChFP-tagged α-syn in Neuro 2A cell lysate (corresponding to a cell density of 4 × 106cell per ml) upon exposure of the cells to exogenous α-syn fibrils or ribbons (2 μM monomeric concentration, for example, particle concentration of 0.25 and 2.2 nM for fibrils and ribbons, respectively) in the presence of the indicated concentrations of proteinase K (μg ml−1). The samples were analysed on 15% SDS–PAGE. The degradation profile of ChFP-tagged α-syn puncta seeded by α-syn fibrils (a) differs very significantly from that of ChFP-tagged α-syn puncta seeded by α-syn ribbons (b). Both patterns differ from that of ChFP-tagged α-syn from untreated Neuro 2A cells (c). The immunoreactivity of HSPA8 was used as a loading control (d). The molecular mass markers (in kilodaltons) are indicated. Figure 6: The two α-syn polymorphs imprint their intrinsic architecture to endogenous α-syn upon its recruitment. Western blot analysis of the degradation profiles of the reporter ChFP-tagged α-syn in Neuro 2A cell lysate (corresponding to a cell density of 4 × 10 6 cell per ml) upon exposure of the cells to exogenous α-syn fibrils or ribbons (2 μM monomeric concentration, for example, particle concentration of 0.25 and 2.2 nM for fibrils and ribbons, respectively) in the presence of the indicated concentrations of proteinase K (μg ml −1 ). The samples were analysed on 15% SDS–PAGE. The degradation profile of ChFP-tagged α-syn puncta seeded by α-syn fibrils ( a ) differs very significantly from that of ChFP-tagged α-syn puncta seeded by α-syn ribbons ( b ). Both patterns differ from that of ChFP-tagged α-syn from untreated Neuro 2A cells ( c ). The immunoreactivity of HSPA8 was used as a loading control ( d ). The molecular mass markers (in kilodaltons) are indicated. Full size image The exceptional protein plasticity of α-syn has led to the protein-chameleon concept [44] , according to which it adopts different structures depending on its environment. Such a concept implies that it can assemble into a variety of structurally distinct high-molecular weight particles. Here we generated two homogeneous different high-molecular weight assemblies from the same precursor α-syn. The two forms exhibit fundamental differences in their building principles. The packing of α-syn molecules within the two polymorphs is different, the amino acid residues involved into rigid structures within α-syn fibrils and ribbons are not the same and the number of amino acids involved into highly ordered structures differs significantly in α-syn fibrils and ribbons, indicating that the intermolecular interactions within the two polymorphs are different. The behaviour of the variant α-syn A30P that is involved in a familial form of the Parkinson’s disease illustrates well the differences in the packing of α-syn molecules within the fibrils and the ribbons. Indeed, while capable of assembling into fibrils, A30P α-syn is incapable of forming ribbons, certainly because of the involvement of amino-acid residue 30 in the packing of α-syn molecules within the ribbons as suggested by the solid-state NMR data. Overall, the polymorphism we observe certainly reflects the ability of α-syn to populate multiple conformational states, allowing the establishment of different intermolecular interactions at the origin of distinct high-molecular weight assemblies that grow indefinitely by incorporation of monomers in a given conformational state. In prions, strains are believed to be the consequence of the ability of a given high molecular assembly of the prion protein to recruit and imprint its intrinsic structure to the newly incorporated prion molecule. Thus, the indefinite growth of different stable prion nuclei is highly dependent on the conformations prion molecules populate in solution and their ability to interact with nuclei’s ends. We demonstrate here that α-syn fibrils and ribbons propagate faithfully their intrinsic structure by recruiting under their respective assembly experimental conditions soluble α-syn molecules in conformations that allow sustained α-syn fibrils or ribbons growth. Interestingly however, under conditions where α-syn ribbons form, the soluble precursor of α-syn fibrils does not appear to be populated, whereas other conformations are, thus leading to unfaithful elongation of α-syn fibrils into ribbons. These findings suggest that strain stability is mostly dependent on the conformational ensembles that precursor soluble polypeptides populate. Besides the differences in the packing of their building blocks and growth and amplification properties, prion strains vary in their tropism for cells as revealed by the strain-specific physiopathological patterns they cause and variations in recipient animal survival rates. The two α-syn polymorphs we generated exhibit marked differences in their propensities to bind and penetrate cells, their toxicity and seeded aggregation of reporter α-syn aggregation in vivo . The finding that externally applied α-syn fibrils have in vivo a better nucleating activity than α-syn ribbons suggests that α-syn folding intermediates that can be recruited by α-syn fibrils are populated to a higher extent than those that elongate α-syn ribbons in the cells. We also demonstrated that α-syn fibrils and ribbons imprint their intrinsic architecture to endogenous α-syn upon its recruitment in vivo . This yield α-syn aggregates within the cells that persist to different extents. The fascinating observations that different α-syn polymorphs have different binding and penetration propensities within cells and different toxicity, together with the finding that they have the ability to induce the aggregation of reporter α-syn in vivo by imprinting their intrinsic architecture to the reporter endogenous α-syn leading to differences in the persistence rates of the assemblies, provide a molecular basis for the heterogeneous group of neurodegenerative disorders caused by α-syn aggregation. These disorders include Parkinson’s disease, dementia with Lewy bodies, pure autonomic failure and multiple system atrophy whose molecular signature is the deposition of α-syn assemblies in selective populations of neurons and glial cells within the human brain. While there is yet no evidence for the presence of different α-syn strains in human, the finding that the two polymorphs bind to different extents to cultured cells albeit with similar kinetics may account for the spatiotemporal spread of α-syn assemblies within the brain described by Braak et al . [25] , [45] Indeed, Lewy neurites and Lewy bodies first appear in the dorsal motor nucleus of the vagal nerve in the brainstem and anterior olfactory structures, then spread stereotypically to large parts of the brain [25] , [45] . This neuropathological progression may thus be the consequence of differences in the tropism of α-syn polymorphs for neuronal cell populations while the assemblies are propagating from one cell to another within the brain. Expression and purification of α-syn The Escherichia coli strain BL21(DE3) (Stratagene, La Jolla, CA, USA) was transformed with the expression vector pET3a encoding wild-type WT α-syn. Recombinant WT α-syn was expressed in E. coli strain BL21(DE3) and purified as previously described [46] , and N15-C13-labelled proteins were produced by pelleting bacteria grown in LB medium to an optical density of 0.8, washing the pellet with M9 medium, suspending the pellet in half the original volume of M9 medium containing 1.75 g of 15 NH 4 Cl, 2.5 g of U- 13 C glucose, 2 mM MgSO 4 , 0.1 mM CaCl 2 and 10 μg thiamine per liter of culture. Cells were further grown for 30 min at 37 °C and α-syn expression was induced by 0.5 mM IPTG for 3 h. α-syn concentration was determined spectrophotometrically using an extinction coefficient of 5960 M −1 cm −1 at 280 nm. Pure α-syn (0.2–0.5 mM) in 50 mM Tris–HCl, pH 7.5, 150 mM KCl was filtered through sterile 0.22-μm filters and stored at −80 °C. Assembly of α-syn into fibrils and ribbons For fibril formation, soluble WT α-syn was incubated in buffer A (50 mM Tris-HCl, pH 7.5, 150 mM KCl) at 37 °C under continuous shaking in an Eppendorf Thermomixer set at 600 r.p.m. Assembly was monitored continuously in a Cary Eclipse spectrofluorimeter (Varian Inc., Palo Alto, CA, USA) in the presence of Thioflavin T (15 μM) in 1 × 1 cm cuvettes under agitation (100 r.p.m.) using a magnetic stir bar (6 × 3 mm) with excitation wavelength set at 440 and emissions wavelengths set at 440 and 480 nm, and an averaging time of 1 s. For ribbon formation, WT α-syn was dialysed 16 h against 1,000 volume of buffer B (5 mM Tris-HCl pH 7.5) at 4 °C, then incubated at 37 °C under continuous shaking in an Eppendorf Thermomixer set at 600 r.p.m. Assembly was monitored by the measurement of the scattered light at 440 nm. Alternatively, the amount of protein remaining in the supernatant after sedimentation at 35,000 g was determined by measurement of the absorbance at 280 nm in a Hewlett Packard 8453 diode array spectrophotometer. The nature of the oligomeric species was assessed using a Jeol 1400 (Jeol Ltd.)TEM following adsorption of the samples onto carbon-coated 200-mesh grids and negative staining with 1% uranyl acetate. The images were recorded with a Gatan Orius CCD camera (Gatan). The ability of α-syn assemblies to bind Congo red was assessed as follows: α-syn fibrils and ribbons were incubated for 1 h with 100 μM Congo Red (Sigma-Aldrich, St Louis, MO, USA) in 20 mM Tris buffer (pH 7.5). The polymers were then sedimented at 20 °C in a TL100 Tabletop Beckman ultracentrifuge (Beckman Instruments, Inc., Fullerton, CA, USA) at 25,000 g for 30 min. The pellets were washed four times using an equal volume of water. Following resuspension of the pellets an aliquot was placed on a glass coverslip and imaged immediately or allowed to dry. Samples were viewed in bright field and cross-polarized light by polarization microscopy using a Leica (MZ12.5) microscope equipped with cross-polarizers (Leica Microsystems, Ltd., Heerbrugg, Switzerland). Disassembly of α-syn fibrils Disassembly of α-syn fibrils was induced by incubating the cuvette at 4 °C in wet ice. Disassembly was monitored using a sedimentation assay. Aliquots (90 μl) were withdrawn at different time intervals from the disassembly reaction and spun at 40,000 g for 30 min at 20 °C in a TL100 tabletop ultracentrifuge (Beckman). The proteins within the supernatant and pellet fractions were analysed by SDS–PAGE and quantified following staining/destaining using the ImageJ software (National Institute of Health, available at rsb.info.nih.gov/ij ). Determination of α-syn fibrils and ribbons concentrations The length heterogeneity of α-syn fibrils and ribbons was reduced by sonication for 20 min on ice in 2-ml Eppendorf tubes in a VialTweeter powered by an ultrasonic processor UIS250v (250 W, 2.4 kHz; Hielscher Ultrasonic, Teltow, Germany) set at 75% amplitude, 0.5 s pulses. The sedimentation velocities of α-syn fibrils and ribbons were measured. The sedimentation boundaries were analysed with the software Sedfit, using the least squares boundary modelling ls–g*(s), which is most suited for heterogeneous mixtures of large particles ( Supplementary Fig. S5 ). This yielded a distribution of particles with sedimentation coefficients ranging from 50 to 150S for α-syn ribbons, from 100 to 1,000S for α-syn fibrils, centred on species that have sedimentation coefficient of ~90S and 375S for α-syn ribbons and fibrils, respectively ( Supplementary Fig. S5A ), corresponding to particles that have a molecular weight of ~11,500 kDa, for example, made of ~800 α-syn molecules (12,000 kDa/14.5 kDa) for α-syn ribbons, ~102,000 kDa, for example, made of ~7,000 α-syn molecules (10,2000, kDa/14.5 kDa) for α-syn fibrils. Thus, at the working concentration of 20 μM, the overall particle concentrations of α-syn ribbons and fibrils are 20 μM/~800 that is, ~0.02 μM, 20 μM/~7,000 that is, ~0.003 μM for α-syn ribbons and fibrils, respectively, given that 100% of α-syn is assembled in ribbons or fibrils at a steady state, as 100% of the protein is found in the pellet fraction upon centrifugation of the samples. We also performed length distribution measurements on α-syn ribbons and fibrils using quantitative TEM ( Supplementary Fig. S5B ). The length and width of ~2,360 fibrils and ~1,790 ribbons were measured using ~50 quantitative negatively stained electron micrographs. The length distribution reveals that the fibrils are ~23 nm wide and ~155 nm long, whereas the ribbons are ~20 nm wide and ~140 nm long ( Supplementary Fig. S5C ). The fibrils were assimilated to cylinders, the average fibril volume was calculated and the number of monomers within a fibril was estimated to ~3,600 α-syn monomers using the equation: where V fib is the volume of a cylinder ( x nm long with y nm diameter), V aa is the volume on average of an amino acid (1.28 × 10 −28 m 3 ) and N , the number of residues within the polypeptide chain (140). Ribbons were assimilated to rectangles and their height (6 nm) was derived from cryo-electron microscopy observations. The number of monomers within a ribbon was estimated using the equation: where V rib is the volume of a rectangle ( x nm long, y nm wide and z nm high), V aa is the volume on average of an amino acid (1.28 × 10 −28 m 3 ) and N , the number of residues within the polypeptide chain (140). Thus, a 140-nm long, 20-nm wide and 6-nm high ribbon contains ~950 α-syn monomers. Analytical ultracentrifugation Sedimentation velocity measurements were carried out using a Beckman Optima XL-A ultracentrifuge equipped with UV-visible detection system using an AN60-Ti four-hole rotor and cells with two-channel 12-mm path-length centerpieces. Samples of α-syn fibrils and ribbons (400 μl) were spun at 5,000 r.p.m. (1818 g ) at 20 °C. Sample displacement profiles were obtained by recording the absorbance at 280 nm every 5 min. Sedimentation coefficient ls–g*(s) distributions were determined using the software Sedfit [47] , [48] . For each experimental condition used, the partial specific volume, the buffer viscosity and density were calculated with the software Sednterp. For all the measurements, the sedimentation coefficient values were corrected to s 20,w (standard solvent conditions in water at 20 °C). Fourier transform infrared spectroscopy α-syn fibrils and ribbons were centrifuged for 20 min at 16,000 g and at 4 °C then extensively washed through four cycles of resuspension and sedimentation with D2O. The spectra were recorded on a JASCO 660 Plus Fourier transform infrared spectroscopy (FTIR) spectrometer equipped with a liquid nitrogen-cooled MCT detector. The background consisted of D 2 O and water vapour. A total of 512 interferograms were collected with a resolution of 2 cm −1 . The sample chamber was continuously purged with dry nitrogen. All the spectra were baseline-corrected, smoothed and normalized prior to further data processing. The amide I (1,600–1,700 cm −1 ) band of the spectra was fitted using a Gaussian species model centred at 1,628, 1,648, 1,661, 1,680 cm −1 (ref. 49 ). During the fitting procedure the peak height was free, whereas the width at half-height was maintained at <25 cm −1 . Proteolytic digestions α-syn fibrils and ribbons (1.4 mg ml −1 ) in 20 mM Tris-HCl, pH 7.5, 1 mM EGTA were treated at 37 °C by Proteinase K (3.8 μg ml −1 ) (Roche). Aliquots were removed at different time intervals following addition of the protease and transferred into Eppendorf tubes maintained at 90 °C containing sample buffer (50 mM Tris-HCl, pH 6.8, 4% SDS, 2% ß-mercaptoethanol, 12% glycerol and 0.01% bromophenol blue) to arrest immediately the cleavage reaction. After incubation of each tube for 10 min at 90 °C, the samples were processed to monitor the time course of α-syn cleavage by Tricine–SDS–polyacrylamide (15%) gel electrophoresis (PAGE) [50] . X-ray fibre diffraction α-syn fibrils and ribbons were desalted by centrifugation at 50,000 r.p.m. for 2 h at 4 °C in a TL100 using a TLA 100.3 rotor. The pellets were resuspended twice in distilled water. Twenty microlitres of pelleted polymers were introduced into a 1-mm diameter glass capillary and dehydrated at room temperature for 2 days. X-ray fibre diffraction patterns were collected at room temperature on the X06DA beamline at the Swiss Light Source, Paul Scherrer Institut, Villigen, Switzerland. The detector used is a MAR225 detector with a 1-Å wavelength, an 8–10–12 cm sample to detector distance, beam size 50 × 80μm. Images were converted using Image J software, re-centred and circularly averaged using a homemade C-programme. Circular profiles of each reflection were extracted to assess reflection types: equatorial, meridional or cross reflection. Characterization of α-syn assemblies α-syn fibrils and ribbons (400 ng), in 20 mM Tris–HCl, pH 7.5, were spotted onto duplicate nitrocellulose membranes. The membranes were blocked in 5% dried skimmed milk and probed with fibril-specific FILA-1 (ref. 32 ) or pan-α-syn antibodies at a concentration of 2 ng μl −1 . Following wash with TBST, the membranes were incubated with HRP-conjugated swine-anti-rabbit secondary antibody (DAKO, Copenhagen, Denmark) for 1 h at room temperature. Proteins were visualized using ECL reagents (Pierce, USA). Cell culture Human neuroblastoma SH-SY5Y cells (ECACC; Sigma-Aldrich), and murine neuroblastoma Neuro 2a cells (ATCC) were cultured at 37 °C in humidified air with 5% CO 2 in Dulbecco’s modified Eagle’s medium Neuro 2a cells) or Dulbecco’s modified Eagle’s Medium/Ham’s nutrient mixture F-12 (SH-SY5Y cells) containing 10% fetal bovine serum, 2 mM glutamine, 100 units ml −1 penicillin and 100 μg ml −1 streptomycin. All materials used for cell culture were from PAA Laboratoires GmbH (Pasching, Austria). Differentiation of SH-SY5Y cells was achieved by treatment of the cells for 1 week with 15 μM retinoic acid (Sigma) that was renewed every 2 days. Cell viability assays The toxicity of α-syn fibrils and ribbons was assessed by cell survival counting and by the MTT reduction inhibition assay. Equal numbers of cells lifted by 0.5 mM EDTA were incubated in suspension in the presence of increasing concentrations of α-syn assemblies for 20 min. Cells were then replated on Petri dishes and cultured for 24 h in the presence of added α-syn. The surviving adherent cells were then lifted by EDTA and their number was determined in the presence of trypan blue in six independent experiments using a hemocytometer. Cell viability data were analysed using two-sample, two-tailed independent Student’s t -tests. For the MTT assay, cells were plated at a density of 1,500 cells per well on 96-well plates in 100 μl of culture medium. After 48 h, the medium was exchanged with 100 μl of fresh medium containing 10 μM of α-syn fibrils and ribbons. Controls samples were prepared with the addition of identical volumes of buffer. After 24 h of incubation, the cells were incubated for another 2 h with 100 μl of serum-free Dulbecco’s modified Eagle’s medium without phenol red, containing 0.5 mg ml −1 MTT. Then, 100 μl of cell lysis solution (20% SDS, 50% N,N-dimethylformamide) was added to each well, and the samples were incubated at 37 °C to allow complete lysis. The absorbance of the formazan was measured at 570 nm in a FlexStation3 microplate reader (Molecular Devices, Sunnyvale, CA, USA). ROS measurement Intracellular ROS levels were determined using the fluorescent probe CellROX Orange Reagent from Life Technologies. Subconfluent differentiated SH-SY5Y cells cultured on 15 μ-Slide eight-well Ibidi (Biovalley) were incubated with 0.2 nM α-syn fibrils or ribbons for 1–6 h. After treatment, the cells were loaded with 5 μM CellROX Orange Reagent for 30 min at 37 °C, washed with serum-free, phenol red-free Dulbecco’s modified Eagle’s Medium/Ham’s nutrient mixture F-12 and immediately imaged on a Zeiss Axio Observer Z1 epifluorescence microscope equipped with an Incubator XLmulti S1 RED LS (Carl Zeiss) and an Orca-R2 camera (Hamamatsu). The cellular fluorescence was quantified using the ImageJ software, after background subtraction for each image. Apoptotic marker measurements Three apoptotic markers were measured. Early apoptosis was assessed by annexin V binding to the cell membranes and caspase-3 activity quantification. Late apoptosis was documented by measurement of nuclear DNA fragmentation. For caspase-3 activity, cells treated for 24 h with α-syn fibrils and ribbons were lysed in 20 mM Tris-HCl, pH 7.5, 250 mM NaCl, 2 mM EDTA, 0.1% Triton X-100 and 1 mM DTT. Extracts obtained from equal numbers of cells were incubated for 2 h at 37 °C in the presence of 50 μM N-acetyl-DEVD-7-amino-4-trifluoromethylcoumarin fluorogenic substrate (Enzo Life Sciences) in 50 mM HEPES-KOH, pH 7.0, 10% glycerol, 0.1% 3-((3-cholamidopropyl)-dimethylammonium)-1-propane sulphonate, 2 mM EDTA, 10 mM DTT. The fluorescence of the aminofluorocoumarin formed upon cleavage of the substrate by caspase-3 was measured in the Cary Eclipse spectrofluorimeter with excitation and emission wavelengths set at 400 and 505 nm, respectively. The translocation of phosphatidylserine (PS) to the outer surface of the cell membrane, an event associated with the onset of apoptosis, was assessed using phycoerythrin-labelled annexin V (annexin V-PE) binding to the cell membrane [51] . After treatment with α-syn fibrils or ribbons, differentiated SH-SY5Y cells were harvested and co-labelled with annexin V-PE (eBioscience) and 2 μg ml −1 of the membrane-impermeable DNA dye 7-amino-actinomycin D (7-AAD) (Biomol), an indicator of cell membrane integrity, in 10 mM Hepes-NaOH, pH 7.4, 140 mM NaCl, 2.5 mM CaCl 2 for 20 min at room temperature. The cells were then analysed by flow cytometry using a Guava EasyCyte Plus System (Guava Technologies), and the percentage of annexin V-positive/7-AAD-negative cells (early apoptotic cells) was quantified. Quantification of DNA fragmentation was performed by terminal deoxynucleotidyl transferase-mediated dUTP nick-end labelling (TUNEL) assay. SH-SY5Y adherent cells exposed to α-syn fibrils or ribbons, lifted with trypsin/EDTA and washed with PBS, were fixed with 1% paraformaldehyde for 20 min at 4 °C. The TUNEL reactions were carried out by the DeadEND Fluorometric TUNEL assay System (Promega), according to the manufacturer’s instructions. The nuclei were counterstained with 5 μg ml −1 propidium iodide (Sigma). The percentage of apoptotic (TUNEL-positive) nuclei was quantified by flow cytometry using a MoFlo Astrios Cell Sorter (Beckman Coulter). The cell population was gated by forward and side scatter and at least 10,000 cells were recorded. The geometric means of the gated population was determined using Summit 5.0 software (Beckman Coulter). Apoptotic nuclei of adherent cells were also imaged by epifluorescence microscopy after counterstaining with Hoechst 33258 (1 μg ml −1 ). α-syn interactions with phospholipid unilamellar vesicles Lipids were purchased from Avanti Polar Lipids (Alabaster, AL, USA). Vesicles containing 1,2-dioleoyl phosphatidylserine (DOPS), 1,2-dioleoyl phosphatidylcholine (DOPC), 1,2-dioleoyl phosphatidylglycerol (DOPG) and porcine brain total lipid extract were dissolved in chloroform and dried in glass tubes under a gentle nitrogen stream. The lipid films were hydrated at 10 mg ml −1 in 50 mM Hepes (pH 7.5), subjected to five freeze–thaw cycles of 2 min each, subjected to sonication for 20 min and centrifuged at 10,000 g for 10 min. For membrane association, 8 nM of α-syn fibrils or ribbons were incubated with phospholipid vesicles (6.25 mM lipids) for 30 min at room temperature in 200 μl of 50 mM Hepes (pH 7.5), and fractionated on an 80–60–10% sucrose gradient. The protein–lipid mixture was adjusted to 80% sucrose by addition of a freshly prepared 100% sucrose in 50 mM Hepes, pH 7.5 solution (800 μl). One mililitre of 60% sucrose was layered over this solution and 0.5 ml of 10% sucrose was layered on the top of the 60% sucrose solution. The tubes were spun at 40,000 r.p.m. in a Beckman SW60 rotor for 16 h at 15 °C in an Optima L90K Beckman ultracentrifuge. Incubation of α-syn fibrils or ribbons did not affect their intrinsic structures as assessed from electron microscopy observation and limited proteolysis analysis ( Supplementary Fig. S11 ). After ultracentrifugation, nine fractions with increasing sucrose concentration were collected from the top of the gradient and processed for 10% Tricine–SDS–PAGE to assess the distribution of the protein throughout the gradient. Following Coomassie Blue staining, the protein content of each fraction was quantified using the ImageJ software. For calcein release, the lipid films were resuspended in 50 mM Hepes pH 7.5 containing 60 mM calcein (Sigma) and treated as described above. The excess non-encapsulated calcein was removed by gel-filtration on PD-10 desalting columns (GE Healthcare). Calcein-loaded lipid vesicles were incubated in 50 mM Hepes pH 7.5 in the presence of 0.7 nM α-syn fibrils or ribbons in 1 cm path-length cuvettes with magnetic stirring in the Cary Eclipse spectrofluorimeter with the excitation and emission wavelengths set at 490 nm and 520 nm, respectively. Calcein is self-quenched in the vesicle aqueous core and its α-syn-mediated leakage to the external medium can be monitored over time (30 min) as an increase in fluorescence. The extent of calcein release was expressed as a fraction of the maximum release due to complete vesicle disruption upon addition of 0.1% Triton X-100 at the end of each experiment. Cell sorting and epifluorescence microscopy imaging α-syn fibrils and ribbons in PBS were labelled by addition of 2 molar excess of the aminoreactive fluorescent dye Alexa Fluor 488 carboxylic acid, succinimidyl ester (Invitrogen). Labelling was performed following the manufacturer’s recommendations. Unreacted dye was removed by three cycles of sedimentation and suspension of the fibrils or ribbons in PBS. To monitor the binding of α-syn polymorphs to the cell membrane, SH-SY5Y cells lifted with EDTA were washed in ice-cold PBS containing 1 μg ml −1 of propidium iodide. At time zero, Alexa Fluor 488-labelled α-syn fibrils or ribbons (0.1 nM) were added to the cells (10 6 cells per ml) and analysis was performed using a using a MoFlo Astrios Cell Sorter (Beckman Coulter). The dead time was estimated to 20 s. The cell population was gated by forward and side scatter and at least 10,000 cells were recorded. The geometric means of the gated population was determined using Summit 5.0 software (Beckmann). To monitor intracellular free Ca 2+ levels, subconfluent cells were loaded for 30 min with 5 μM of the fluorescent dye Fluo-4-acetoxymethyl ester (Fluo-4-AM) (Invitrogen) in the presence of 0.02% ( w / v ) Pluronic Acid F127 and 2.5 mM of the organic anion-transport inhibitor probenecid (Invitrogen). The cells were then washed and incubated with varying concentrations of α-syn fibrils or ribbons in serum-free, phenol red-free Dulbecco’s modified Eagle’s Medium/Ham’s nutrient mixture F-12, and imaged over time on the Axio Observer Z1 epifluorescence microscope (Zeiss). Images were acquired every 20 s for 30 min at 37 °C in humidified air with 5% CO 2 . The fluorescence was quantified using the ImageJ software, after background subtraction for each image. The fluorescence is expressed as a fraction of the maximum fluorescence recorded upon addition of ionomycin to the cells. In vivo nucleation activities of a-syn assemblies To assess the ability of α-syn fibrils and ribbons to induce the aggregation of endogenous, soluble α-syn, Neuro 2a cells stably expressing ChFP–α-syn, grown on poly- L -lysine-coated coverslips, selected and maintained at 400 μg ml −1 of G418 were exposed to Alexa Fluor 488-labelled α-syn fibrils and ribbons (0.01 nM and 0.1 nM particles concentrations, 0.05 μM precursor soluble protein concentration) for 4 h. Cells on coverslips were washed with PBS and fixed with 4% paraformaldehyde. Cells with ChFP puncta were scored from at least 300 cells in randomly selected fields by epifluorescence microscopy. The amount of cell-associated Alexa Fluor 488-labelled α-syn fibrils and ribbons was determined by direct measurement of fluorescence in a population of cells exposed to 0.1–0.01 nM Alexa Fluor 488-labelled α-syn fibrils and ribbons compared with the fluorescence of Alexa Fluor 488 standards. To generate the stable cell lines, a plasmid encoding α-syn-CherryFP was made by PCR amplification of WT α-syn cDNA and subcloning into pCDN 3.1 vector (already containing ChFP insert) between the Hin dIII and Bgl II sites. Transfection was performed using Lipofectamin2000 following the manufacturer instruction. Stables cell lines expressing α-syn-CherryFP were selected using neomycin (G418) for 3 weeks, and sorted on the basis of their levels of expression by FACS (FACSAria III, BD Biosciences). Digestion of cell extracts and western blot analysis Neuro 2A cells (2 × 10 6 ) grown on 60 cm 2 Petri dishes were treated with 7 ml of medium containing α-syn fibrils or ribbons (2 μM monomeric concentration, for example, particle concentration of 0.25 and 2.2 nM for fibrils and ribbons, respectively). The cells were washed and recovered in PBS at a final density of 4 × 10 6 cell per ml. They were sonicated thrice for 10 s on ice at an intensity of 5 using a Branson sonifier (model 150) equipped with a 3-mm microtip, and the lysate was flash-frozen in liquid nitrogen. Aliquots (20 μl) of cell lysate exposed or not to α-syn fibrils or ribbons were treated with increasing concentrations of PK (0.01–1 μg ml −1 ) for 20 min at 37 °C. The digestion reaction was stopped by addition of PMSF to a final concentration of 1 mM and the samples were immediately denatured by the addition of preheated (95 °C) sample buffer (50 mM Tris–HCl, pH 6.8, 4% SDS, 2% ß-mercaptoethanol, 12% glycerol and 0.01% bromophenol blue). After a 5 min incubation at 95 °C, the samples were analysed on 15% SDS–PAGE followed by western blotting using rabbit polyclonal antibody directed against human full-length wild-type α-syn and imaged on a Fuji LAS3000 imager. How to cite this article: Bousset, L. et al . Structural and functional characterization of two alpha-synuclein strains. Nat. Commun. 4:2575 doi: 10.1038/ncomms3575 (2013).